miR-191 and miR-135 are required for long-lasting spine remodelling associated with synaptic long-term depression Activity-dependent modification of dendritic spines, subcellular compartments accommodating postsynaptic specializations in the brain, is an important cellular mechanism for brain development, cognition and synaptic pathology of brain disorders. NMDA receptor-dependent long-term depression (NMDAR-LTD), a prototypic form of synaptic plasticity, is accompanied by prolonged remodelling of spines. The mechanisms underlying long-lasting spine remodelling in NMDAR-LTD, however, are largely unclear. Here we show that LTD induction causes global changes in miRNA transcriptomes affecting many cellular activities. Specifically, we show that expression changes of miR-191 and miR-135 are required for maintenance but not induction of spine restructuring. Moreover, we find that actin depolymerization and AMPA receptor exocytosis are regulated for extended periods of time by miRNAs to support long-lasting spine plasticity. These findings reveal a miRNA-mediated mechanism and a role for AMPA receptor exocytosis in long-lasting spine plasticity, and identify a number of candidate miRNAs involved in LTD. Dendritic spines are tiny protrusions from dendritic shafts where the majority of excitatory synapses in the central nervous system are located [1] . The size and geometry of dendritic spines are coupled to synaptic strength [2] , [3] , and are modulated by synaptic activity to accompany the functional change of synapses during synapse development and synaptic plasticity [4] . Activity-induced changes in spines occur in both directions. For instance, long-term depression (LTD) of synaptic transmission is usually associated with spine shrinkage and loss, while long-term potentiation (LTP) of synaptic transmission is characterized by spine enlargement and formation [5] , [6] . The changes in dendritic spines during synaptic plasticity can be maintained for prolonged periods of time [5] . Long-lasting modification of dendritic spines is an important cellular mechanism for information storage in the brain [7] , [8] . N-methyl-D-aspartate (NMDA) receptor-dependent LTD (NMDAR-LTD) is a form of synaptic plasticity important for learning and memory. LTD impairment in mice caused by knockout of NMDA receptor subunits or inhibition of NMDA receptor signalling pathways is associated with cognitive deficits such as dysfunctions in spatial learning, working memory and behavioural flexibility [9] , [10] , [11] . Induction of NMDAR-LTD is accompanied by spine shrinkage and loss. The mechanisms underlying the structural and functional plasticity in LTD overlap partially. For instance, they both require NMDA receptors, calcineurine and actin depolymerization, but AMPA receptor endocytosis and protein phosphatase 1 are only involved in synaptic depression [5] , [12] , [13] . Despite intensive study of synaptic plasticity, however, the molecular mechanisms underlying spine remodelling associated with LTD, especially long-term maintenance of changes in spines, are still largely unclear. microRNAs (miRNAs) are short, non-coding RNAs that bind to mRNAs to inhibit translation and/or promote mRNA degradation by imperfect base-pairing between the seed region in miRNAs (usually nucleotides 2–8 at the 5′ end) and the miRNA-binding site in the 3′ untranslated region (3′ UTR) of target mRNAs [14] . Each miRNA can potentially target to hundreds of distinct mRNAs, and thousands of genes are regulated by miRNAs. miRNAs are increasingly recognized as key regulators of gene expression and have been found to play important roles in diverse cellular processes such as the differentiation and development of cells [15] , [16] . miRNAs are crucial for proper brain function. Of the >1,000 miRNAs identified in mammals, hundreds are expressed in the brain [17] , [18] . miRNA loss in mice due to deficientexpression of Dicer or DGCR8, two essential components of the miRNA biogenesis pathway [15] , leads to alterations in synaptic protein expression, synaptic transmission, dendritic spines, learning and memory [19] , [20] . Several miRNAs, such as miR-134, miR-125, miR-138, miR-132, miR-29 and miR-188, regulate the morphogenesis of dendritic spines [16] , [21] , [22] . The expression of miRNAs is changed during LTP and metabotropic glutamate receptor-dependent LTD, and is regulated by BDNF, which contributes to long-lasting modification of synaptic function [23] , [24] . Despite the demonstrated importance of miRNAs, however, the function of the vast majority of miRNAs expressed in the brain have yet to be elucidated, due in part to the limited capacity of traditional experimental techniques and the large number of miRNAs and their target genes. The question of whether or not miRNAs play a role in spine remodelling associated with LTD also remains open. Here using next-generation deep sequencing and bioinformatic analyses, we identify miRNAs differentially expressed in hippocampal neurons undergoing LTD, and genes and cellular processes potentially targeted by them. Moreover, by examining the functions of miR-191 (downregulated) and miR-135 (upregulated) in hippocampal neurons, we show that both up- and downregulation of protein synthesis resulting from changes in miRNA transcriptomes are required for persistent and delayed, but not for the initiation of, spine restructuring in LTD. We demonstrate specifically that miR-191 and miR-135 contribute to spine remodelling by regulating the expression of their target genes tropomodulin 2 and complexin-1/2, respectively. In addition, we find that actin depolymerization and AMPA receptor exocytosis are regulated by miRNAs for prolonged periods of time in long-lasting spine plasticity. This study provides a catalogue of miRNAs, genes and cellular processes potentially involved in spine plasticity associated with LTD, demonstrates that miRNAs are crucial regulators of gene expression to orchestrate cellular processes essential for long-lasting structural changes of synapses, and identifies a novel function of AMPA receptor exocytosis in spine plasticity. Changes in the miRNA transcriptome during NMDAR-LTD To determine whether miRNAs are involved in spine remodelling associated with LTD, we first used next-generation deep sequencing to systematically interrogate the change in miRNA expression following induction of NMDAR-LTD in the mouse hippocampus. To induce LTD, hippocampal slices from mice (17–19 days old) were treated with NMDA (30 μM, 5 min). NMDA treatment induces ‘chemical LTD’, which shares molecular mechanisms with electrical stimulation-induced LTD and causes long-lasting synaptic depression and spine loss in most synapses of the slice [13] , [25] , [26] . Consistent with reported studies, after NMDA treatment we observed a persistent decrease in field excitatory postsynaptic potentials (fEPSP) of CA1 neurons (mean±s.e.m. : 20.3±4.0% of baseline at 10 min, 55.4±5.4% of baseline at 90 min, 62.3±5.6% of baseline at 2 h after stimulation; n =10 slices for each group; Supplementary Fig. 1 ). At 90 min after LTD induction, the CA1 region was removed for RNA extraction and preparation of miRNA sequencing libraries. A total of eight libraries (four NMDA-treated and four sham-treated controls) were sequenced by using an Illumina GAII analyser. On average, 0.92 million reads were generated from each library, 52.65% of which were mapped to mature miRNAs. From the total 3,660,602 mapped reads, 438 mature miRNAs were identified ( Fig. 1a,b ). The number of miRNAs detected by our deep sequencing is in line with previous reports that ~300 miRNAs are expressed in the rodent brain [17] , [27] . 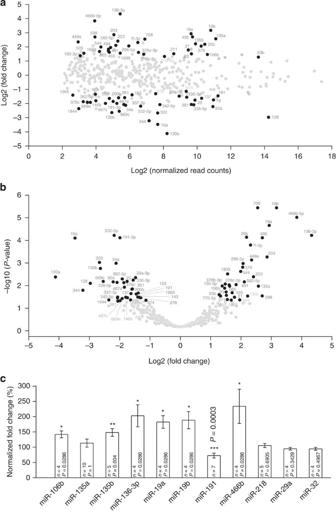Figure 1: The change of miRNA transcriptomes in the hippocampus following LTD induction. Hippocampal slices were prepared from mice (17–19 days old) and either sham-treated or treated with NMDA (30 μM, 5 min) to induce chemical LTD. miRNAs were isolated at 90 min after NMDA treatment for deep sequencing (a,b) or qRT–PCR (c). (a) The fold change (log2 scale) of each miRNA species is plotted against its normalized read number (log2 scale). (b) TheP-value (log10 scale) of each miRNA species is plotted against its fold change (log2 scale). (c) qRT-PCR analysis of miRNA expression.n=4–10 experiments for each miRNA. Inaandb, miRNAs withP-values <0.05 are represented by dark circles. Inc, data are presented as mean±s.e.m.; Mann–WhitneyU-test is used for statistical analysis; *P<0.05, **P<0.01, ***P<0.005. Figure 1: The change of miRNA transcriptomes in the hippocampus following LTD induction. Hippocampal slices were prepared from mice (17–19 days old) and either sham-treated or treated with NMDA (30 μM, 5 min) to induce chemical LTD. miRNAs were isolated at 90 min after NMDA treatment for deep sequencing ( a , b ) or qRT–PCR ( c ). ( a ) The fold change (log2 scale) of each miRNA species is plotted against its normalized read number (log2 scale). ( b ) The P -value (log10 scale) of each miRNA species is plotted against its fold change (log2 scale). ( c ) qRT-PCR analysis of miRNA expression. n =4–10 experiments for each miRNA. In a and b , miRNAs with P -values <0.05 are represented by dark circles. In c , data are presented as mean±s.e.m. ; Mann–Whitney U -test is used for statistical analysis; * P <0.05, ** P <0.01, *** P <0.005. Full size image The fold change and P -value of individual miRNAs are illustrated in Fig. 1 . The fold changes are independent of the count of expression tags ( Fig. 1a ), suggesting that our deep sequencing was unbiased on miRNA abundance. The P -value was computed by controlling the false discovery rate (FDR) for multiple hypothesis testing [28] , and a P -value cutoff of 0.05 was applied to select differentially expressed miRNAs ( Fig. 1b ). A total of 70 miRNAs were changed in expression after LTD induction (34 upregulated, 36 downregulated; Fig. 1a,b ). To validate the deep-sequencing result with an independent assay and preparation, we measured the expression change of several miRNAs in cultured hippocampal neurons using quantitative real-time PCR (qRT-PCR). Neurons (DIV17) were treated with NMDA (30 μM, 5 min) and harvested at 90 min after stimulation for RNA isolation and qRT-PCR. The expression of miR-191 decreased, that of miR-106b, miR-135b, miR-136-3p, miR-19a, miR-19b and miR-466b increased, and that of miR-218, miR-29a and miR-32 remained unaltered following NMDA treatment ( Fig. 1c ). The expression level of miR-135a slightly increased, but not to a statistically significant level ( P =1.00). These qRT-PCR results are largely consistent with our findings using deep sequencing. Taken together, these results indicate that following LTD induction the miRNA transcriptome changes substantially, suggesting that miRNAs may play roles in the structural and functional plasticity of synapses. Genes and cellular processes targeted by changed miRNAs miRNAs exert their cellular functions mainly by regulating translation of mRNAs. Each type of miRNA can potentially regulate hundreds of mRNA transcripts, and in most cases, a single mRNA is targeted by multiple miRNA species. To obtain a comprehensive view of the impact of miRNA transcriptome changes on cell physiology, we conducted the miR-gene-gene ontology (GO) enrichment analysis [27] for miRNAs differentially expressed in LTD. To focus on miRNAs that are likely to have significant effects on gene expression, we analysed only those with read counts >30 in all samples. Up- and downregulated miRNAs were analysed in separate groups. The complete lists of enriched genes and GO terms are shown in Supplementary Data 1 and 2 . Some enriched GO terms are related to the regulation of synaptic functions and dendritic spines, such as ‘synaptic transmission’, ‘actin filament-based process’, ‘cytoskeletal protein binding’, ‘regulation of phosphorylation’ and ‘small GTPase-mediated signal transduction’. These GO terms along with their corresponding miRNAs are illustrated in Supplementary Fig. 2 and Supplementary Data 2 . Our findings from these analyses suggest that in neurons undergoing LTD, differentially expressed miRNAs regulate many different cellular processes involved in the structural and functional remodelling of synapses. miR-191 and miR-135 regulate prolonged spine remodelling To examine how altered miRNA expression affects synaptic modification following LTD induction, we conducted time-lapse imaging in cultured hippocampal neurons. In this test, we focused on miR-191 and miR-135, which target to genes and GO terms implicated in the remodelling of dendritic spines and synaptic plasticity. For instance, miR-191 targets tropomodulin 2, which regulates actin dynamics, and the GO terms ‘cytoskeletal protein binding’ and ‘synaptic transmission’. Likewise, miR-135 targets complexin-1 and -2, which regulate AMPA receptor trafficking, and the GO terms ‘cytoskeleton organization’, ‘regulation of MAPK cascade’ and ‘actin filament-based process’ ( Supplementary Fig. 2 , Supplementary Data 1 and 2 ) [29] , [30] , [31] , [32] . Our deep sequencing shows that while miR-191 is downregulated, both miR-135a and miR-135b, the two isoforms of miR-135 that target to same genes, are upregulated after LTD induction. To counteract their changes in expression during LTD, we transfected hippocampal neurons (DIV14) with constructs expressing miR-191 or miR-135 sponge that sequesters endogenous miR-135a/b and increases the expression of its confirmed targets complexin-1 and -2 ( Supplementary Figs 3a,b and 4c ) or antisense oligonucleotides against miR-135a/b. A construct expressing venus (a mutant of YFP) [33] was co-transfected to visualize dendritic spines. At 3–5 days after transfection, neurons were treated with NMDA (30 μM, 5 min) for LTD induction. Time-lapse confocal microscopy was used to image the same spines of transfected neurons before and at 10, 30 and 90 min after NMDA treatment. NMDA treatment caused rapid shrinkage of spines. By 10 min after stimulation, spine area was reduced by 11.2±3.0% (mean±s.e.m. ; n =8 cells for the sham-treated group, n =15 cells for the NMDA-treated group; Fig. 2 ). The decrease in spine size was progressive and long-lasting. By 90 min after stimulation, spine size was reduced by 24.5±3.8% (mean±s.e.m. ; n =9 cells for the sham-treated group, n =16 cells for the NMDA-treated group) and more spines were retracted ( Fig. 2 ). 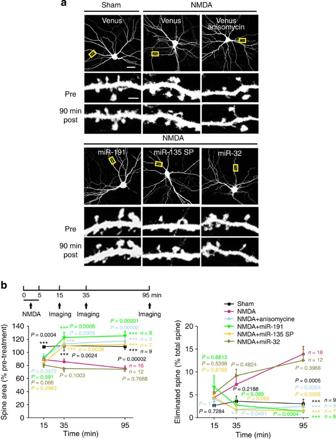Figure 2: miR-191 and miR-135 are essential for long-lasting spine restructuring accompanying LTD. Cultured hippocampal neurons (DIV14) were transfected with the venus construct alone or along with the construct expressing miR-191, miR-32 or sponge against miR-135a and miR-135b. At 3–5 days after transfection, neurons were imaged before and at 10, 30 and 90 min after treatment. Anisomycin (20 μM) was added to the bath solution at 10 min before NMDA treatment (30 μM, 5 min) and present throughout the imaging period. (a) Representative images. Yellow boxes indicate the dendrites in the high-magnification images. (b) Quantification ofa.n=7–16 neurons for each group. Data are presented as mean±s.e.m. Mann–WhitneyUtest was used for statistical analysis of the NMDA-treated, venus-transfected group versus other groups. ***P<0.005. Scale bars, 20 μm in the top image ofa, 5 μm in the high-magnification image ofa. Figure 2: miR-191 and miR-135 are essential for long-lasting spine restructuring accompanying LTD. Cultured hippocampal neurons (DIV14) were transfected with the venus construct alone or along with the construct expressing miR-191, miR-32 or sponge against miR-135a and miR-135b. At 3–5 days after transfection, neurons were imaged before and at 10, 30 and 90 min after treatment. Anisomycin (20 μM) was added to the bath solution at 10 min before NMDA treatment (30 μM, 5 min) and present throughout the imaging period. ( a ) Representative images. Yellow boxes indicate the dendrites in the high-magnification images. ( b ) Quantification of a . n =7–16 neurons for each group. Data are presented as mean±s.e.m. Mann–Whitney U test was used for statistical analysis of the NMDA-treated, venus-transfected group versus other groups. *** P <0.005. Scale bars, 20 μm in the top image of a , 5 μm in the high-magnification image of a . Full size image In cells transfected with the miR-191 construct, the miR-135 sponge construct or antisense oligonucleotides against miR-135, NMDA-induced spine shrinkage at 10 min post-stimulation was comparable to that in control cells ( Fig. 2 , Supplementary Fig. 3c,d ). However, spine size gradually recovered thereafter, and was indistinguishable from sham-treated cells by 30 min after stimulation ( Fig. 2 , Supplementary Fig. 3c,d ). The increase in spine retraction was also abolished by transfection with the miR-191 construct, miR-135 sponge or miR-135 antisense oligonucleotides ( Fig. 2 , Supplementary Fig. 3c,d ). We also transfected neurons with a construct expressing miR-32, whose expression was unaffected by NMDA treatment ( Fig. 1 ), or with scrambled miR-135 oligonucleotides. Neither the size of spines, nor NMDA-induced spine shrinkage and retraction were affected by transfection of the miR-32 construct or scrambled oligonucleotides ( Fig. 2 , Supplementary Fig. 3c,d ). In addition, without NMDA treatment, the size and density of dendritic spines were unaffected by transfection of the miR-191 construct, miR-135 sponge, miR-135 antisense oligonucleotide or the miR-32 construct ( Supplementary Fig. 3e ). These results suggest that the effect of miR-191, miR-135 sponge or antisense oligonucleotides on NMDA-induced spine plasticity is not due to non-specific changes in cell physiology. Taken together, these results indicate that miR-191 inhibits, while miR-135 promotes, NMDA-induced spine retraction and long-lasting spine shrinkage, and therefore suggest that their expression changes in LTD are required for prolonged spine remodelling. Spine remodelling in LTD is translation-dependent As the main function of miRNAs is translational regulation, our findings on miR-191 and miR-135 suggest that protein synthesis might be involved in the modification of spines during LTD. To test this possibility, we tested the effects of the translational inhibitors anisomycin and emetine on NMDA-induced spine remodelling. Prior to NMDA treatment, anisomycin (20 μM) and emetine (20 μM) were added to the bath solution of neurons transfected with a construct expressing venus. In inhibitor-treated cells, spine size was reduced at 10 min post-stimulation with NMDA, but by 30 and 90 min after stimulation, it is comparable to that in sham-treated cells ( Fig. 2 , Supplementary Fig. 3c,d ). The two translational inhibitors also abolished NMDA-induced spine retraction ( Fig. 2 , Supplementary Fig. 3c,d ). By contrast, the transcriptional inhibitor actinomycin D (10 μM) had no effects on NMDA-induced spine shrinkage or retraction ( Supplementary Fig. 3c,d ). These results indicate that translation, but not transcription, is required for NMDA-induced spine elimination and persistent reduction in spine size. Tropomodulin 2 is miR-191’s target and is upregulated in LTD To determine how miR-191 regulates spine remodelling, we looked into its target genes. Among miR-191’s predicted targets, tropomodulin 2 (Tmod2) has two predicted miR-191-binding sites in its 3′UTR and the most total favourable context score for miR-191 recognition [34] , [35] . Moreover, based on our miR-gene-GO enrichment analysis, some GO terms targeted by Tmod2, such as ‘cytoskeletal protein binding’, are closely related to spine remodelling ( Supplementary Figs 2 and 5a , Supplementary Data 2 ). Hence, we tested whether Tmod2 mediates the effect of miR-191 on spine plasticity associated with LTD. First, we tested whether Tmod2 is a true target of miR-191. We generated a reporter construct by inserting the 3′UTR of Tmod2 behind the destabilized mCherry sequence. This reporter construct was transfected into cultured hippocampal neurons (DIV14) along with a plasmid expressing both EGFP and miR-191. At 3 days after transfection, mCherry expression was assessed by measuring the intensity ratio of fluorescence produced by mCherry and EGFP. The expression of mCherry by the reporter construct was greatly reduced by co-transfection with the miR-191 construct, but not a construct expressing miR-135b, which is not predicted to interact with Tmod2, or an EGFP construct expressing no miR-191 ( Fig. 3a,b ). To test whether miR-191 represses mCherry expression through the miR-191-binding sites in the 3′UTR of Tmod2, we mutated the miR-191-binding sites in the reporter construct, and found that mCherry expression by the mutated reporter construct was no longer affected by transfection of the miR-191 plasmid ( Fig. 3a,b ). These results indicate that the 3′UTR of Tmod2 confers translational control by miR-191. 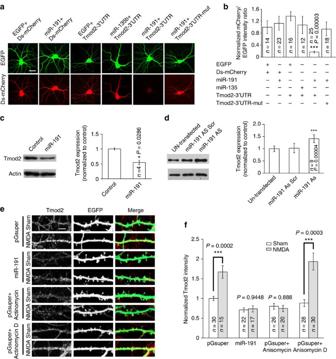Figure 3: Tmod2 is a physiological target of miR-191 and increased in expression by NMDA treatment. Cultured hippocampal neurons (a,b,e,f) and cortical neurons (c,d) were transfected with designated constructs at DIV14 or transduced with lentivirus at DIV7, and imaged or harvested for immunoblotting at DIV17. (a) Representative images of neurons co-transfected with the miRNA and reporter constructs. (b) Quantification ofa. (c) Western blots of cell lysates from neurons transduced with the miR-191 or control virus;n=4 experiments. (d) Western blots of cell lysates from neurons transfected with the miR-191 antisense oligonucleotides or scrambled oligonucleotides;n=4–9 experiments for each condition. (e) Representative images of dendrites transfected with the miR-191 construct or the control plasmid. (f) Quantification ofe.n=12–30 cells for each group inbandf. Data are presented as mean±s.e.m. Mann–WhitneyU–test was used for statistical analysis. ***P<0.005. Scale bars, 20 μm ina, 5 μm ine. Figure 3: Tmod2 is a physiological target of miR-191 and increased in expression by NMDA treatment. Cultured hippocampal neurons ( a , b , e , f ) and cortical neurons ( c , d ) were transfected with designated constructs at DIV14 or transduced with lentivirus at DIV7, and imaged or harvested for immunoblotting at DIV17. ( a ) Representative images of neurons co-transfected with the miRNA and reporter constructs. ( b ) Quantification of a . ( c ) Western blots of cell lysates from neurons transduced with the miR-191 or control virus; n =4 experiments. ( d ) Western blots of cell lysates from neurons transfected with the miR-191 antisense oligonucleotides or scrambled oligonucleotides; n =4–9 experiments for each condition. ( e ) Representative images of dendrites transfected with the miR-191 construct or the control plasmid. ( f ) Quantification of e . n =12–30 cells for each group in b and f . Data are presented as mean±s.e.m. Mann–Whitney U –test was used for statistical analysis. *** P <0.005. Scale bars, 20 μm in a , 5 μm in e . Full size image To test whether miR-191 also regulates endogenous Tmod2 expression, cultured cortical neurons were transduced with lentivirus expressing miR-191, or transfected with antisense oligonucleotides against miR-191. Tmod2 expression was analysed by immunoblotting. The miR-191 virus reduced, while antisense oligonucleotides increased Tmod2 expression ( Fig. 3c,d and Supplementary Fig. 4a ). These results confirm that Tmod2 is a physiological target of miR-191. Next, we tested whether Tmod2 expression is changed during LTD. Cultured hippocampal neurons were treated with NMDA (30 μM, 5 min), and stained with the Tmod2 antibody at 90 min after stimulation. In cells transfected with the control plasmid, NMDA treatment caused an increase in Tmod2 expression, and this increase was induced at the translational but not transcriptional level, as the translational inhibitor anisomycin inhibited it, but the transcriptional inhibitor did not ( Fig. 3e,f ). To test whether miR-191 contributes to the change in Tmod2 expression, we transfected neurons with the miR-191 construct to compensate for NMDA-induced reduction in miR-191 expression. miR-191 transfection abolished NMDA-induced changes in Tmod2 expression ( Fig. 3e,f ). These data indicate that NMDA-induced decreases in miR-191 expression results in enhanced expression of Tmod2. Taken together, these findings indicate that Tmod2 is a physiological target of miR-191 and that reduced miR-191 expression during LTD leads to increased expression of Tmod2. Tmod2 is essential for spine plasticity associated with LTD Having demonstrated that Tmod2 is a target of miR-191 and is upregulated following LTD induction, we next examined its role in spine plasticity. To this end, we generated a construct expressing siRNAs against Tmod2. The efficacy and specificity of Tmod2 siRNAs were tested against exogenously and endogenously expressed Tmod2 in COS-7 cells and primary hippocampal neurons, respectively ( Supplementary Fig. 5b–e and Supplementary Fig. 4d ). Cultured hippocampal neurons (DIV14) were transfected with the highly effective and specific Tmod2 siRNA (siRNA-4), treated with NMDA (30 μM, 5 min), and imaged before and after NMDA treatment. As measured at 10, 30 and 90 min after NMDA stimulation, the size of spines and the number of eliminated spines in Tmod2 siRNA transfected and sham-treated neurons were comparable ( Fig. 4 ). Transfection of the Tmod2 siRNA construct did not change the basal level of spine size or density ( Supplementary Fig. 5f,g ). These results indicate that Tmod2 is required for NMDA-induced spine shrinkage and elimination. 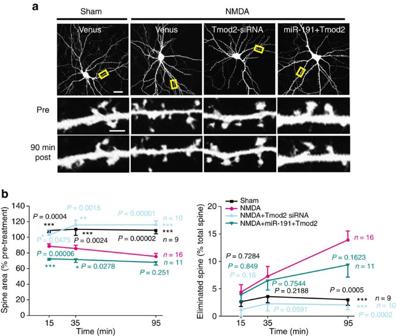Figure 4: Tmod2 mediates the effect of miR-191 on spine remodelling during LTD. Cultured hippocampal neurons (DIV14) were transfected with the venus construct alone or along with the designated constructs. At 3–5 days after transfection, neurons were imaged before and at 10, 30 and 90 min after treatment. (a) Representative images. Yellow boxes indicate the dendrites in the high-magnification images. (b) Quantification ofa.n=8–16 neurons for each group. Data are presented as mean±s.e.m. Mann–WhitneyU-test was used for statistical analysis of the NMDA-treated, venus-transfected group versus other groups. *P<0.05, **P<0.01, ***P<0.005. Scale bars, 20 μm in the top image, 5 μm in the high-magnification image. Figure 4: Tmod2 mediates the effect of miR-191 on spine remodelling during LTD. Cultured hippocampal neurons (DIV14) were transfected with the venus construct alone or along with the designated constructs. At 3–5 days after transfection, neurons were imaged before and at 10, 30 and 90 min after treatment. ( a ) Representative images. Yellow boxes indicate the dendrites in the high-magnification images. ( b ) Quantification of a . n =8–16 neurons for each group. Data are presented as mean±s.e.m. Mann–Whitney U -test was used for statistical analysis of the NMDA-treated, venus-transfected group versus other groups. * P <0.05, ** P <0.01, *** P <0.005. Scale bars, 20 μm in the top image, 5 μm in the high-magnification image. Full size image To test whether Tmod2 mediates miR-191 function in LTD, we transfected hippocampal neurons (DIV14) with the miR-191-expressing construct along with a construct expressing Tmod2, and stimulated these cells with NMDA (30 μM, 5 min) at 3 days after transfection. The size and density of spines were not changed by co-transfection of the Tmod2 siRNA and the miR-191 construct ( Supplementary Fig. 5f,g ). While long-lasting spine shrinkage and spine elimination induced by NMDA treatment were both blocked in miR-191-transfected cells ( Fig. 2 ), co-transfection of the Tmod2 with the miR-191 construct restored these changes ( Fig. 4 ). These results indicate that miR-191 restricts spine plasticity by limiting the expression of Tmod2. To test whether other miR-191 target genes also regulate spine remodelling, we co-transfected hippocampal neurons (DIV14) with the miR-191 construct and a construct expressing EGR1 (a reported miR-191 target) [36] . NMDA-induced spine shrinkage and elimination were indistinguishable in miR-191- and EGR1-co-transfected and miR-191-overexpressing cells ( Supplementary Fig. 6 ). Hence, unlike Tmod2, EGR1 does not contribute to the function of miR-191 in NMDA-induced spine remodelling. Taken together, these findings indicate that in LTD increased Tmod2 expression resulting from a reduction in miR-191 is required to maintain spine changes. Tmod2 modifies actin filaments in LTD Tmod2 is a neuron-specific member of the tropomodulin family [37] . Tropomodulins are actin filament-pointed end-capping proteins that regulate the dynamics, length and amount of actin filaments (F-actin) [29] . Since actin depolymerization is promoted by LTD induction and underlies spine shrinkage [5] , [31] , Tmod2 may also play a role in actin regulation during LTD. To test this possibility, we transfected cultured hippocampal neuron (DIV14) with a construct expressing the Tmod2 siRNA construct, and stained F-actin with phalloidin. In neurons transfected with the control plasmid, NMDA treatment caused a reduction in the F-actin content ( Fig. 5 ). Tmod2 siRNA-transfected cells, however, contained comparable levels of F-actin, whether or not they were treated with NMDA ( Fig. 5 ). Likewise, transfection of the miR-191 construct also blocked NMDA-induced F-actin change ( Fig. 5 ), and this effect of miR-191 was obliterated by co-transfection with a construct expressing Tmod2 ( Fig. 5 ). By contrast, transfection with the miR-135b construct or miR-135 antisense oligonucleotides had no effect on NMDA-induced F-actin reduction ( Fig. 5 ). These results indicate that Tmod2 is required for NMDA-induced actin reorganization and for the effect of miR-191 downregulation on F-actin. 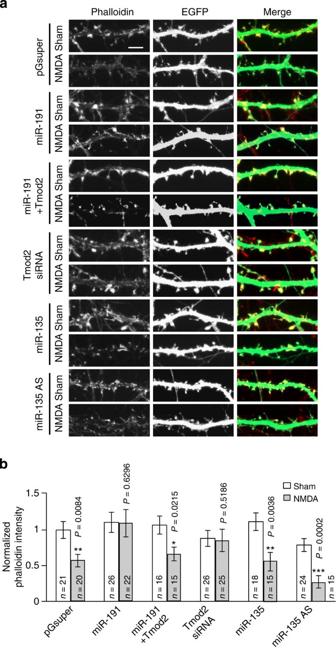Figure 5: Tmod2 is required for NMDA-induced reduction in actin filament. Cultured hippocampal neurons (DIV14) were transfected with the designated constructs. At DIV17, neurons were stained with rhodamine phalloidin at 90 min after NMDA treatment (30 μM, 5 min). (a) Representative images of transfected dendrites. (b) Integrated fluorescence intensity of phalloidin per μm2dendrite area normalized to the sham-treated group.n=15–26 neurons for each group. Data are presented as mean±s.e.m. Mann–WhitneyU-test was used for statistical analysis. *P<0.05, **P<0.01, ***P<0.005. Scale bar, 5 μm. Figure 5: Tmod2 is required for NMDA-induced reduction in actin filament. Cultured hippocampal neurons (DIV14) were transfected with the designated constructs. At DIV17, neurons were stained with rhodamine phalloidin at 90 min after NMDA treatment (30 μM, 5 min). ( a ) Representative images of transfected dendrites. ( b ) Integrated fluorescence intensity of phalloidin per μm 2 dendrite area normalized to the sham-treated group. n =15–26 neurons for each group. Data are presented as mean±s.e.m. Mann–Whitney U -test was used for statistical analysis. * P <0.05, ** P <0.01, *** P <0.005. Scale bar, 5 μm. Full size image miR-135 regulates complexin-1/2 for spine remodelling in LTD miR-135 targets both complexin-1 and -2 ( Supplementary Fig. 3a,b and Supplementary Fig. 4c ), which are 86% identical at the amino-acid level in rats and perform redundant functions [38] . In addition, our miR-gene-GO enrichment analysis found that complexin-1 and -2 are annotated by GO terms related to spine morphogenesis, such as ‘nervous system development’ ( Supplementary Data 2 , Supplementary Fig. 5a ), suggesting that they might be involved in spine plasticity. Hence, we tested whether complexins mediate the promoting effect of miR-135 on spine remodelling during LTD. If complexins are, in fact, miR-135 effectors in LTD, it is likely that NMDA treatment will alter complexin expression. To test this possibility, we treated cultured cortical neurons (DIV17) with NMDA (30 μM, 5 min) and assessed complexin expression by immunoblotting with an antibody against both complexin-1 and -2. The expression of both complexin-1 and complexin-2 was decreased by NMDA treatment, and this decrease was abolished by transfection with the miR-135 antisense oligonucleotides prior to NMDA treatment ( Fig. 6a,b and Supplementary Fig. 4b ). These results indicate that by upregulating miR-135, NMDA treatment decreases the expression of complexin-1 and -2. 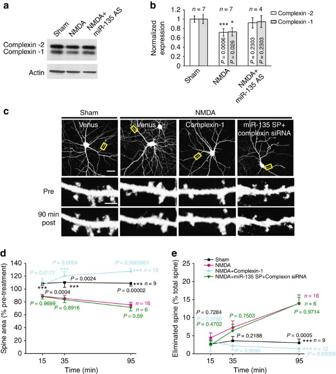Figure 6: Complexins mediate the effect of miR-135 on spine remodelling during LTD. Cultured cortical neurons (DIV14) were transfected with antisense oligonucleotides against miR-135 and treated with NMDA, followed by immunoblotting against complexin-1 and -2 inaandb. Inc–e, cultured hippocampal neurons (DIV14) were transfected with the venus construct alone or along with the designated construct. At 3–5 days after transfection, neurons were imaged before and at 10, 30 and 90 min after treatment. (a) Representative blots. (b) Quantification ofa.n=4–7 experiments for each condition. (c) Representative images. Yellow boxes indicate the dendrites in the high-magnification images. (d,e) Quantification ofc.n=6–16 neurons for each group indande. Data are presented as mean±s.e.m. Mann–WhitneyU-test was used for statistical analysis of the NMDA-treated, venus-transfected group versus other groups. *P<0.05, ***P<0.005. Scale bars, 20 μm in the top image ofc, 5 μm in the high-magnification image ofc. Figure 6: Complexins mediate the effect of miR-135 on spine remodelling during LTD. Cultured cortical neurons (DIV14) were transfected with antisense oligonucleotides against miR-135 and treated with NMDA, followed by immunoblotting against complexin-1 and -2 in a and b . In c – e , cultured hippocampal neurons (DIV14) were transfected with the venus construct alone or along with the designated construct. At 3–5 days after transfection, neurons were imaged before and at 10, 30 and 90 min after treatment. ( a ) Representative blots. ( b ) Quantification of a . n =4–7 experiments for each condition. ( c ) Representative images. Yellow boxes indicate the dendrites in the high-magnification images. ( d , e ) Quantification of c . n =6–16 neurons for each group in d and e . Data are presented as mean±s.e.m. Mann–Whitney U -test was used for statistical analysis of the NMDA-treated, venus-transfected group versus other groups. * P <0.05, *** P <0.005. Scale bars, 20 μm in the top image of c , 5 μm in the high-magnification image of c . Full size image To test whether the expression change of complexins is required for spine remodelling, we transfected hippocampal neurons (DIV14) with the venus construct along with a construct expressing complexin-1 to compensate for diminished complexin expression induced by NMDA treatment. At all examined time points after NMDA stimulation, spine size and elimination were comparable in complexin-1-transfected cells and sham-treated controls ( Fig. 6c–e ). Transfection of the complexin-1 construct left the basal level of spine size and density intact ( Supplementary Fig. 7a,b ). These results indicate that the reduction in complexin expression is required for NMDA-induced spine shrinkage and elimination. To test whether complexins mediate the effect of miR-135 on spine remodelling, we transfected hippocampal neurons (DIV14) with a construct expressing siRNAs against both complexin-1 and -2 ( Supplementary Figs 4e and 7c,d ) along with the miR-135 sponge construct or miR-135 antisense oligonucleotides. Co-transfection of the complexin-1 construct and the miR-135 sponge construct or miR-135 antisense oligonucleotides did not change the baseline of spine size and density ( Supplementary Fig. 7a,b ). While NMDA-induced spine elimination and long-lasting spine shrinkage were blocked by miR-135 sponge or antisense oligonucleotides ( Fig. 2 , Supplementary Fig. 8 ), these changes were restored in cells co-transfected with the complexin siRNA construct and miR-135 sponge or antisense oligonucleotides ( Fig. 6c–e , Supplementary Fig. 8 ). These results show that regulation of complexin expression by miR-135 promotes spine remodelling. To test whether other miR-135 targets also contribute to NMDA-induced spine remodelling, we co-transfected hippocampal neurons (DIV14) with the miR-135 sponge construct and a construct expressing siRNAs against Rap2, which is also a target gene of miR-135 ( Supplementary Figs 3a,b, 4c,f and 7e,f ). Transfection of the Rap2 siRNA construct left the effect of miR-135 sponge on NMDA-induced spine shrinkage and elimination unchanged ( Supplementary Fig. 8 ), indicating that Rap2 does not mediate the function of miR-135 in spine remodelling. Taken together, these results indicate that complexin-1 and -2 are the targets of miR-135, responsible for its function in NMDA-induced spine remodelling. Reduced complexin expression alters AMPA receptor exocytosis Complexin-1 and -2 are SNARE complex-binding proteins and regulate both pre- and post-synaptic exocytosis [30] , [39] . Although the role of postsynaptic exocytosis in LTD has yet to be examined, it has been shown to regulate spine size during LTP [40] . To determine the mechanism by which complexin contributes to spine remodelling, we explored the possibility that complexins regulate postsynaptic exocytosis in LTD. First, we tested whether LTD induction alters dendritic exocytosis. Exocytosis of postsynaptic membrane was assessed by monitoring exocytosis of the AMPA receptor subunit GluA1 using fluorescence recovery after photobleaching (FRAP). Cultured hippocampal neurons (DIV14) were transfected with a DsRed construct (for visualization of neuronal morphology) along with a construct expressing GluA1 tagged with a pH-sensitive form of EGFP (Super Ecliptic pHluorin, SEP) that displays fluorescence only when it is present on the cell surface [41] , [42] , [43] . At 3–5 days after transfection, neurons were treated with NMDA (30 μM, 5 min). At 30 min after NMDA treatment, a small dendritic segment (25–30 μm) was photobleached to eliminate >95% SEP fluorescence, and images were taken every 2–10 min thereafter. After photobleaching, SEP fluorescence in sham-treated neurons gradually recovered, with a recovery time constant ( τ ) of 21.6±3.0 min (mean±s.e.m., n =12 cells; Fig. 7 ). By contrast, NMDA treatment greatly slowed GluA1 recovery after photobleaching ( τ =105.2±11.8 min, mean±s.e.m., n =7 cells, P =0.00008 versus sham-treated controls, U -test; Fig. 7 ). These results indicate that AMPA receptor exocytosis is inhibited by NMDA treatment. 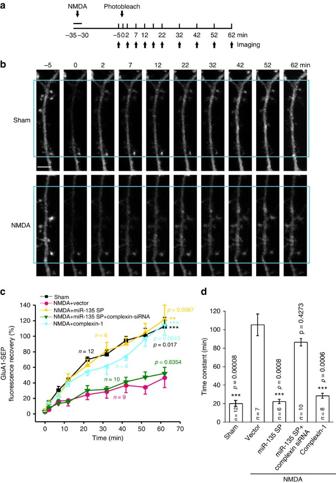Figure 7: Inhibition of GluA1 exocytosis by miR-135 following NMDA treatment. Cultured hippocampal neurons (DIV14) were transfected with the DsRed and GluA1-SEP constructs, along with the designated plasmids. At 3–5 days after transfection, neurons were treated with NMDA (30 μM, 5 min), photobleached and imaged at various time points as indicated. (a) Schematic drawing of the experimental design. (b) Representative images. Dendritic regions in the blue boxes were photobleached. (c) Fluorescence recovery curve of each group. (d) Time constant of FRAP.n=5–12 neurons for each group. Data are presented as mean±s.e.m. Mann–WhitneyU-test was used for statistical analysis of the NMDA-treated, DsRed and GluA1-SEP-transfected group versus other groups. **P<0.01, ***P<0.005. Scale bars, 10 μm. Figure 7: Inhibition of GluA1 exocytosis by miR-135 following NMDA treatment. Cultured hippocampal neurons (DIV14) were transfected with the DsRed and GluA1-SEP constructs, along with the designated plasmids. At 3–5 days after transfection, neurons were treated with NMDA (30 μM, 5 min), photobleached and imaged at various time points as indicated. ( a ) Schematic drawing of the experimental design. ( b ) Representative images. Dendritic regions in the blue boxes were photobleached. ( c ) Fluorescence recovery curve of each group. ( d ) Time constant of FRAP. n =5–12 neurons for each group. Data are presented as mean±s.e.m. Mann–Whitney U -test was used for statistical analysis of the NMDA-treated, DsRed and GluA1-SEP-transfected group versus other groups. ** P <0.01, *** P <0.005. Scale bars, 10 μm. Full size image To test whether miR-135 plays a role in changing AMPA receptor exocytosis, we transfected hippocampal neurons (DIV14) with the miR-135 sponge construct or miR-135 antisense oligonucleotides to counteract NMDA-induced upregulation of miR-135, then measured GluA1 exocytosis. After NMDA treatment, GluA1 exocytosis occurred faster in sponge ( τ =22.3±2.4 min, mean±s.e.m., n =6 cells, P =0.0082 versus NMDA-treated controls, U -test; Fig. 7 ) or antisense oligonucleotides ( τ =21.3±2.4 min, mean±s.e.m., n =10 cells, P =0.0004 versus NMDA-treated controls, U -test; Supplementary Fig. 9 ) transfected cells than in control plasmid-transfected cells. These results indicate that miR-135 inhibits postsynaptic exocytosis following NMDA treatment. Next, we tested whether complexins contribute to NMDA-induced retardation of exocytosis. Hippocampal neurons (DIV14) were transfected with a complexin-1-expressing construct, and treated with NMDA (30 μM, 5 min) at 3–5 days after transfection. GluA1 exocytosis was measured at 30 min after NMDA treatment using FRAP. In the complexin-1 construct-transfected cells, the recovery of GluA1 after photobleaching was faster than in control plasmid-transfected cells, and comparable to that in sham-treated cells ( τ =30.2±2.8 min, mean±s.e.m., n =8 cells, P =0.0006 versus NMDA-treated controls; P =0.12 versus sham-treated cells, U -test; Fig. 7 ), indicating that reduced complexin expression induced by NMDA treatment slows GluA1 exocytosis. To test whether the effect of miR-135 on GluA1 exocytosis is mediated by complexins, we transfected hippocampal neurons with the complexin siRNA construct along with the miR-135 sponge construct or miR-135 antisense oligonucleotides. In the co-transfected cells, GluA1 exocytosis after NMDA treatment was far less than in cells transfected with the miR-135 sponge construct or miR-135 antisense oligonucleotides alone, and comparable to that in NMDA-treated controls ( Fig. 7 , Supplementary Fig. 9 ). By contrast, basal GluA1 exocytosis without NMDA treatment was not affected by miR-135 or complexin-1 ( Supplementary Fig. 10 ). These results indicate that miR-135 regulates AMPA receptor exocytosis in NMDA-treated neurons by suppressing complexin expression. Taken together, these results indicate that postsynaptic exocytosis was decreased by NMDA treatment, and that this decrease is attributable to the repression of complexin expression by miR-135. miR-191 and miR-135 are essential for LTD induction Having delineated the function of miR-191 and miR-135 in spine plasticity associated with LTD, we proceeded to test whether they also play roles in the depression of synaptic transmission. Cultured hippocampal slices were transduced with lentivirus expressing miR-191 or miR-135 sponge. At 5 days after transduction, LTD was induced in the CA1 region by stimulating the Schaffer collateral pathway (1 Hz, 15 min). In control virus-transduced cells, fEPSPs were decreased by the stimulation (mean±s.e.m. : 68.9±2.0% of baseline at 10 min, 64.7±6.1% of baseline at 90 min and 62.7±4.3% of baseline at 2 h after stimulation; n =6 slices; Fig. 9). By contrast, LTD was greatly reduced in cells transduced with the miR-191 or miR-135 sponge virus (mean±s.e.m. : 91.5±7.0% ( P =0.041 versus control), 101.0±4.9% ( P =0.0021 versus control), 101.0±6.4% ( P =0.0043 versus control) and 95.7±7.4% ( P =0.0043 versus control) of baseline for miR-191; 81.9±3.0% ( P =0.0022 versus control), 88.0±2.8% ( P =0.026 versus control), 93.5±6.7% ( P =0.0087 versus control) and 87.5±2.8% ( P =0.0022 versus control) of baseline for miR-135 at 10, 30, 90 and 120 min post-stimulation, respectively. n =6 slices for each group, U -test; Fig. 8 ). These results indicate that the induction of LTD requires proper expression levels of miR-191 and miR-135. 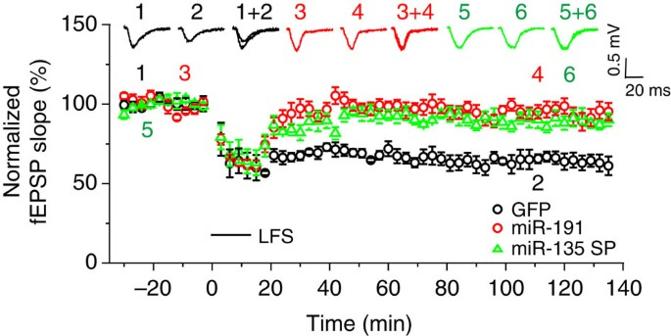Figure 8: miR-191 and miR-135 are involved in LTD induction. Cultured hippocampal slices were transduced with lentivirus expressing miR-191 or miR-135 sponge. At 5 days after transduction, LTD was induced in CA1 neurons by low-frequency stimulation (900 pluses at 1 Hz). fEPSP slopes normalized to the pre-stimulation baseline were plotted as mean±s.e.m.n=6 slices for each group. Figure 8: miR-191 and miR-135 are involved in LTD induction. Cultured hippocampal slices were transduced with lentivirus expressing miR-191 or miR-135 sponge. At 5 days after transduction, LTD was induced in CA1 neurons by low-frequency stimulation (900 pluses at 1 Hz). fEPSP slopes normalized to the pre-stimulation baseline were plotted as mean±s.e.m. n =6 slices for each group. Full size image Both pri- and mature miR-191 and miR-135b are changed in LTD To explore the mechanisms by which miR-191 and miR-135 are changed in LTD, we assessed the levels of pri- and mature miR-191 and miR-135b at various time points after NMDA treatment. Hippocampal neurons (DIV17) were treated with NMDA (30 μM, 5 min) and harvested at 10, 30, 60 and 90 min after NMDA stimulation. Pri- and mature miRNAs were analysed using qRT–PCR. The expression of both mature and pri-miR-191 was reduced by NMDA treatment ( Fig. 9a ). Likewise, both mature and pri-miR-135b were changed by NMDA treatment ( Fig. 9b ). The elevation of mature and pri-miR-135b, however, started earlier than the decrease in mature and pri-miR-191 ( Fig. 9a,b ), suggesting that the expression changes in these two miRNAs might be induced by different mechanisms. 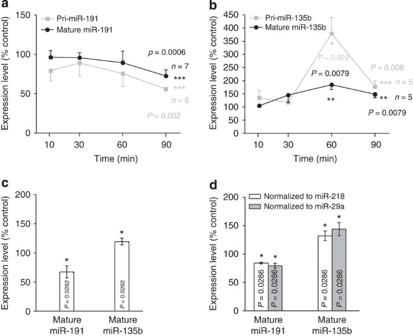Figure 9: miR-191 and miR-135 are modulated at both transcriptional and post-transcriptional levels in LTD. Cultured hippocampal neurons were treated with NMDA (30 μM, 5 min) alone (a,b) or along with actinomycin (c), and collected at indicated time points for qRT-PCR analysis (a–c). Cultured cortical neurons were treated with NMDA (30 μM, 5 min) and used for CLIP assay at 90 min after treatment (d). (a) Time course of NMDA-induced changes in pri- and mature miR-191;n=4–7 experiments for each time point. (b) Time course of NMDA-induced changes in pri- and mature miR-135b;n=4–5 experiments for each time point. (c) The effect of actinomycin on NMDA-induced changes in mature miR-191 and miR-135b;n=7 experiments for each condition. (d) The change in miR-191 and miR-135b associated with RISC;n=4 experiments for each condition. Data are shown as mean±s.e.m. Mann–WhitneyU-test was used for statistical analysis. *P<0.05; **P<0.01, ***P<0.005. Figure 9: miR-191 and miR-135 are modulated at both transcriptional and post-transcriptional levels in LTD. Cultured hippocampal neurons were treated with NMDA (30 μM, 5 min) alone ( a , b ) or along with actinomycin ( c ), and collected at indicated time points for qRT-PCR analysis ( a – c ). Cultured cortical neurons were treated with NMDA (30 μM, 5 min) and used for CLIP assay at 90 min after treatment ( d ). ( a ) Time course of NMDA-induced changes in pri- and mature miR-191; n =4–7 experiments for each time point. ( b ) Time course of NMDA-induced changes in pri- and mature miR-135b; n =4–5 experiments for each time point. ( c ) The effect of actinomycin on NMDA-induced changes in mature miR-191 and miR-135b; n =7 experiments for each condition. ( d ) The change in miR-191 and miR-135b associated with RISC; n =4 experiments for each condition. Data are shown as mean±s.e.m. Mann–Whitney U -test was used for statistical analysis. * P <0.05; ** P <0.01, *** P <0.005. Full size image The changes in the pri form of miR-191 and miR-135b after LTD induction indicate that these miRNAs are regulated at the transcriptional level. To test whether they are also regulated at post-transcriptional levels in LTD, we treated hippocampal neurons (DIV17) with the transcriptional inhibitor actinomycin D (10 μM) along with NMDA. Despite the presence of actinomycin D, NMDA treatment still altered the levels of mature miR-191 and miR-135b ( Fig. 9c ), suggesting that post-transcriptional processing of these miRNAs are also regulated by NMDA treatment. To test whether NMDA-induced changes in miRNAs have impact on miRNAs incorporated into RISC, we analysed miR-191 and miR-135b associated with RISC by using the cross-linking and immunoprecipitation (CLIP) assay. We transduced primary cortical neurons with lentivirus expressing Flag-tagged argonoute 2 (Ago2, a protein component of RISC). At 10 days after transduction, RISC in transduced neurons was crosslinked by UV irradiation, and then pulled down with an anti-Flag antibody. miRNAs in immunoprecipitated RISC were measured by qRT–PCR using miR-218 and miR-29a (two miRNAs unaffected by NMDA treatment, Fig. 1 ) as controls. We found that the level of miRNA-191 in RISC was decreased, and that of miR-135b was increased ( Fig. 9d ). Taken together, these results indicate that in LTD, miR-191 and miR-135b are regulated at both transcriptional and post-transcriptional levels. NMDA treatment alters dendritic miR-191 and miR-135b Several miRNAs and RISC proteins are found in dendrites where they could locally regulate translation [44] . To test whether miR-191 and miR-135b are localized in dendrites, we assessed their subcellular distribution by using in situ hybridization (ISH). Hippocampal neurons (DIV14) were transfected with the EGFP construct for visualization of dendrites. At 3 days after transfection, locked nucleic acid probes were used for miRNA ISH. miR-191 and miR-135b were detected in both soma and dendrites ( Fig. 10a ). By contrast, the signals of a control probe for the U6 small nuclear RNA were found mainly in the soma, and those of another control probe for miR-215 (which is expressed at a negligible level in hippocampal neurons based on our deep-sequencing analysis) were little ( Fig. 10a ), confirming the specificity of our ISH assay. These results indicate that miR-191 and miR-135b are indeed localized in dendrites. 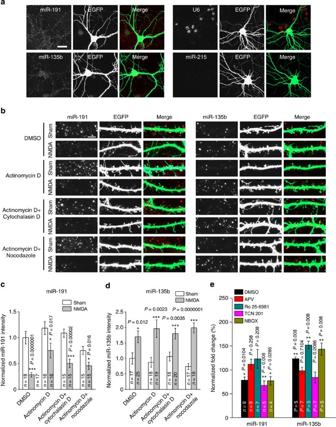Figure 10: miR-191 and miR-135 are regulated locally in dendrites by different NMDAR subunits. Cultured hippocampal neurons were treated with NMDA (30 μM, 5 min) alone or along with various inhibitors as indicated, and used for ISH (a–d) or qRT-PCR at 90 min after treatment (e). (a) Subcellular localization of miR-191 and miR-135b. (b) NMDA-induced changes in miR-191 and miR-135b in dendrites. (c,d) Quantification ofb;n=15–25 neurons for each condition. (e) Regulation of miR-191 and miR-135b by different NMDAR subunits;n=4–9 experiments for each condition. Scale bars: 20 μm for low-magnification (top) and 5 μm for high-magnification images (bottom). Data are shown as mean±s.e.m. Mann–WhitneyU-test was used for statistical analysis. *P<0.05, **P<0.01, ***P<0.005. Figure 10: miR-191 and miR-135 are regulated locally in dendrites by different NMDAR subunits. Cultured hippocampal neurons were treated with NMDA (30 μM, 5 min) alone or along with various inhibitors as indicated, and used for ISH ( a – d ) or qRT-PCR at 90 min after treatment ( e ). ( a ) Subcellular localization of miR-191 and miR-135b. ( b ) NMDA-induced changes in miR-191 and miR-135b in dendrites. ( c , d ) Quantification of b ; n =15–25 neurons for each condition. ( e ) Regulation of miR-191 and miR-135b by different NMDAR subunits; n =4–9 experiments for each condition. Scale bars: 20 μm for low-magnification (top) and 5 μm for high-magnification images (bottom). Data are shown as mean±s.e.m. Mann–Whitney U -test was used for statistical analysis. * P <0.05, ** P <0.01, *** P <0.005. Full size image To test whether dendritic miR-191 and miR-135b are changed in LTD, we treated hippocampal neurons (DIV17, 3 days after transfection with the EGFP construct) with NMDA (30 μM, 5 min). At 90 min after treatment, neurons were fixed for ISH. Notably, miR-191 and miR-135b in dendrites were altered by NMDA treatment ( Fig. 10b–d ). To test whether dentritic miR-191 and miR-135b can be regulated locally in LTD, we treated hippocampal neurons with NMDA along with actiniomycin D (10 μM) to block transcription, and the actin polymerization inhibitor cytochalasin D (10 μM) or the microtubule polymerization inhibitor nocodazole (10 μM) to interfere with intracellular transportation of miRNAs. Dendritic miR-191 and miR-135b were still changed by NMDA treatment when transcription and intracellular trafficking were inhibited ( Fig. 10b–d ). Hence, NMDA treatment can regulate miR-191 and miR-135b locally in dendrites. The dendritic localization of miRNA-191 and miR-135b suggests that they might regulate the expression of their target mRNAs in dendrites. To test this possibility, we first assessed the subcellular localization of Tmod2 and complexin-1 mRNAs. Our ISH assay showed that both Tmod2 and complexin-1 mRNAs were indeed localized in dendrites ( Supplementary Fig. 11a ). We then tested whether expression of dendritic Tmod2 and comlexin-1 were altered in LTD by blocking transcription and intracellular trafficking with actinomycin D, cytochalasin D and nocodazole. Despite the presence of these inhibitors, the expression of both dendritic Tmod2 and complexin-1 and -2 was changed by NMDA treatment ( Supplementary Fig. 11b–e ). These results indicate that the expression of Tmod2 and complexins can be regulated locally in dendrites during LTD. Taken together, these findings indicate that in LTD, the expression changes in miR-191, miR-135b and their targets are caused at least in part by local miRNA processing and translation in dendrites. Different NMDAR subunits regulate miR-191 and miR-135b Having demonstrated the importance of miRNAs in NMDAR-LTD, we went on to test the role played by NMDA receptors in the regulation of miRNAs. We treated hippocampal neurons (DIV17) with NMDA (30 μM, 5 min) along with the NMDAR antagonist AP5 ((2 R )–amino–5–phosphonovaleric acid, 100 μM), and isolated RNA at 90 min after treatment for qRT–PCR analysis of miRNAs. The changes in miR-191 and miR-135b induced by NMDA treatment were blocked by AP5. Hence, NMDAR is essential for the regulation of miRNAs in LTD ( Fig. 10e ). In hippocampal neurons, NMDAR is composed of GluN1 and GluN2 subunits (GluN2A and GluN2B) [45] . GluN1 is an obligate subunit, while GluN2A and GluN2B have different functions. To test which GluN2 subunit regulates miRNAs in LTD, we treated hippocampal neurons (DIV17) with NMDA (30 μM, 5 min) along with the GluN2A antagonist TCN 201 (10 μM) or GluN2B antagonists Ro 25-6891 (3 μM), and isolated RNA at 90 min after treatment. Notably, after NMDA stimulation, the decrease in miR-191 was blocked by GluN2B antagonists (but not the GluN2A antagonist), while the increase in miR-135 was blocked by the GluN2A antagonist (but not GluN2B antagonists) ( Fig. 10e ). By contrast, the AMPA receptor blocker NBQX (2,3-Dioxo-6-nitro-1,2,3,4-tetrahydrobenzo[ f ]quinoxaline-7-sulphonamide, 10 μM) had no effect on NMDA-induced changes in miR-191 and miR-135b ( Fig. 10e ). Taken together, these results indicate that NMDAR is required for the change in miRNA expression associated with LTD, and that GluN2A and GluN2B play different roles in the regulation of miRNAs. In this study, we examined the role of miRNAs in the structural plasticity of dendritic spines in LTD. Using deep sequencing to profile the miRNA transcriptome, we compiled a comprehensive list of miRNAs differentially expressed in LTD. We also employed both computational and experimental approaches to investigate cellular processes regulated by these miRNAs. Our results show that a large number of miRNAs, affecting many different cellular processes, are altered in expression by LTD induction. With live imaging and electrophysiology, we demonstrated experimentally that miR-191 and miR-135 are essential for sustained spine remodelling and induction of synaptic depression in LTD. We also identified the genes and cellular processes targeted by these two miRNAs to modulate spines. While several miRNAs have been shown to regulate dendritic spine morphology, the role of miRNAs in spine plasticity has yet to be examined. Investigation of this question is to some extent hampered by the large number of miRNAs. We tackled this problem by using deep sequencing to screen for candidate miRNAs involved in LTD. The next-generation sequencing technologies have significantly pushed back the limitations of prior transcriptome profiling approaches by greatly improving the throughput, depth of coverage, sensitivity and quantifiability. They are particularly advantageous when analysing miRNAs expressed in the brain, many of which are low- to moderate-abundance transcripts. Our deep-sequencing results reveal notable changes, in both directions, in the miRNA transcriptomes of neurons undergoing LTD. Downregulation of miRNAs is expected to enhance, while the increase in miRNA levels is predicted to suppress translation. Hence, the alteration in miRNA transcriptomes suggests that miRNAs contribute to the bidirectional change of gene expression in LTD. Our findings that a large number of miRNAs are changed in expression after NMDA treatment is in accordance with previous reports that activation of NMDA or metabotropic glutamate receptors has notable effects on miRNA expression [23] , [46] , [47] . In particular, several miRNAs including miR-191, miR-320, miR-106b, miR-203 and miR-21 are identified as differentially expressed miRNAs in both our and in the studies of Kye et al. [46] that stimulate neurons with NMDA. Although in the Kye et al. [46] study, the change in miR-135 expression does not reach a statistically significant level, it shows a trend of increase that is in the same direction as observed in our study. The incomplete overlap in results between our and the Kye et al. [46] study might stem from the differences in cell types and miRNA profiling methods used in the two studies (cultured hippocampal neurons containing all hippocampal regions and quantitative PCR in the Kye et al. [46] study versus the CA1 region from acute hippocampal slices and deep sequencing in our study). We experimentally confirmed that the change in miRNA expression can lead to both increases and decreases in gene expression. For instance, the target of miR-191, Tmod2, is increased, while the targets of miR-135, complexin-1 and -2, are decreased as a consequence of miRNA change. Downregulation of miRNAs is consistent with the accepted notion that the maintenance of synaptic depression is dependent on new protein synthesis [48] , [49] , [50] , and our results that translation is required for long-term stabilization of spine remodelling. Our findings of upregulated miRNAs, however, reveal unexpectedly a new dimension of proteome regulation in LTD—translational inhibition. Importantly, our functional characterization of miR-191 and miR-135 confirms that bidirectional modulation of protein synthesis is essential for spine plasticity. To gain a systematic view of the physiological effects of miRNA transcriptome changes, we used a bioinformatic method, which combines a statistical analysis developed in-house with publicly available computational and experimental data on miRNA targets and gene functions, to predict miRNA targets and cellular processes that are likely to be regulated by differentially expressed miRNAs. This approach facilitates the selection and prioritization of miRNA targets and cellular activities for experimental validation. Results from this analysis suggest that differentially expressed miRNAs regulate a broad range of activities, and that multiple miRNAs might influence the same cellular process concertedly by targeting to its different components. Dendritic spines are actin-rich structures. Actin cytoskeleton is essential to sculpt the shape of spines, and its dynamic rearrangement induced by synaptic activity underlies structural remodelling of spines [31] . LTD-inducing stimulations cause a shift of actin from filamentous actin (F-actin) to globular actin (G-actin) in minutes, and F-actin reduction is required for spine shrinkage [5] , [51] . Activation of the F-actin-severing protein cofilin by dephosphorylation and inactivation of the actin polymerization regulator Arp2/3 complex by protein interaction have been implicated as crucial signalling cascades underlying actin reorganization for spine shrinkage in LTD [52] , [53] . Our findings indicate that the maintenance of F-actin reduction beyond initial spine shrinkage is required to support long-lasting spine remodelling, and that doing so requires the upregulation of Tmod2 by miR-191. AMPA receptor trafficking to and away from postsynaptic membrane is critical for synaptic plasticity [54] , [55] , [56] . In LTD, however, although AMPA receptor endocytosis is a major mechanism of synaptic depression, it is not required for spine shrinkage [12] , [13] . Surprisingly, we found that to stabilize spine shrinkage in LTD, AMPA receptor exocytosis, which is an important means of enhancing synaptic strength in LTP [57] , [58] , [59] , [60] , is inhibied due to miR-135-mediated suppression of complexin expression. Complexin has been indicated in AMPA receptor exocytosis in LTP. The fact that complexin regulates AMPA receptor exocytosis in both LTD and LTP is consistent with the reported interaction between the LTD and LTP pathways [54] , [55] . Our findings that Tmod2 and complexin-1 and -2 are involved in both spine shrinkage and elimination in LTD suggest that these two processes are controlled by overlapping pathways. This model is consistent with the scenario that excessive spine shrinkage can result in spine loss. Our analysis of pri-mRNAs indicates that transcriptional regulation contributes to NMDA-induced changes in mature miRNAs. By using ISH to detect the subcellular localization of miRNAs and blocking transcription and intracellular trafficking, we demonstrated that in LTD, miRNAs can also be regulated at post-transcriptional levels locally in dendrites, consistent with the previous report that pre-miRNAs are indeed localized, and therefore presumably processed, in dendrites [61] . It is conceivable that the dendritic localization of miRNA-processing machinery and its regulation by synaptic transmission allow timely and spatially restricted control of miRNA levels near synapses, thereby facilitating the specificity and efficiency of synaptic activities. Interestingly, both downregulation of miR-191 and upregulation of miR-135b in LTD require NMDAR activity, but are mediated by different GluN2 subunits. It is possible that activation of GluN2A and GluN2B subunits has opposing effects on miRNA biogenesis and/or processing, thereby leading to bidirectional changes in the miRNA transcriptome. Finally, how do cells benefit from using miRNAs to control spine plasticity? While new protein synthesis is required for many forms of synaptic plasticity, such as LTP, LTD and homoeostatic synaptic plasticity [62] , [63] , [64] , different types of synaptic plasticity entail distinct changes in synaptic structure and function. For instance, LTD is characterized by synaptic depression and spine shrinkage, while LTP, its functional opposite, features synaptic potentiation and spine enlargement. Because of their large varieties and base-pairing interaction with mRNAs, miRNAs are well positioned to provide transcript- and stimulation-specific fine-tuning of translation. It is conceivable that combination of gene-specific regulatory mechanisms, such as that dependent on miRNAs, with global translational regulation that has been indicated in synaptic plasticity [64] , can efficiently and precisely modulate the proteome to suit the unique needs of each kind of synaptic plasticity. Animals Male C57BL/6 mice (17–19 days old) were used for deep sequencing, 18–19-day-old Sprague Dawley rat embryos were used for neuronal cultures, and 6–8-day-old Sprague Dawley rats were used for slice cultures. All animal procedures followed the US National Institutes of Health guidelines Using Animals in Intramural Research and were approved by the National Institute of Mental Health Animal Care and Use Committee. DNA constructs and reagents To generate constructs expressing miRNAs, rat pre-miR-135a (primers: 5′-GAAATGGTTTTGAAGTCGT-3′ and 5′-CGTTCCAGAGGCTCTAGTT-3′) and -b (primers: 5′-TTCCTCAGTTTCCTGCTCT-3′ and 5′-CTCTGTGGCTGGTCCTTAG-3′) and pre-miR-191 (primers: 5′-GATGGGCGGGTTCCGGTTT-3′ and 5′-TGGCCCAGTAGTGTTTCTGA-3′) were amplified from genomic DNAs by PCR and cloned into the BglII/HindIII site of the pGSuper vector. The siRNA constructs was made by inserting annealed oligos containing the siRNA sequence against Tmod2 (5′-GGTCAACAAGACCTTGAAA-3′), Complexin-1 and -2 (5′-GGACATGTTCAAGAAGTAA-3′) into the pSuper vector. The cDNAs of Tmod2 and complexin-1 were obtained by RT–PCR and cloned into the GW1 vector. To generate the reporter construct, the 3′UTR of Tmod2 was amplified from rat brain cDNA by PCR and cloned into the pCMV-mCherry-Ds vector behind the mCherry sequence. The miR-191 precursor along with the H1 promoter was amplified from the miR-191-pGsuper construct by PCR (using primers: 5′-GCTGCAGGAATTCGAACG-3′ and 5′-GGTGAGCAAAAACAGGAAGG-3′) and cloned into the pRRLsin.CMV.GFPpre vector for lentivirus production. The miRNA-binding sites in the miR-135 and the miR-215 sponge were designed as reported [65] (miR-135: 5′-TCACATAGGAATTTAAGCCATA-3′; miR-215: 5′-TGTCTGTCAAAGTTAGGTCAT-3′). Ten miRNA-binding sites were inserted into the 3′UTR region of EGFP in the pRRLsin.CMV.GFPpre vector for the production of lentivirus. The following constructs were obtained as gifts: GluR1-SEP (Bo Li, Cold Spring Harbor Laboratory), pRRLsin.CMV.GFPpre (Scott Young, National Institute of Mental Health, National Institutes of Health). The following reagents were obtained commercially: miR-135 and miR-191 antisense oligonucleotide (IDT), NMDA (Sigma-Aldrich), anisomycin (Sigma-Aldrich), Emetine (Sigma-Aldrich), actinomycin D (Sigma-Aldrich), AP5 (Sigma-Aldrich), Ro 25-6891 (Sigma-Aldrich), TCN 201 (Tocris), Cytochalasin (Sigma-Aldrich), Nocodazole (Sigma-Aldrich), NBQX (Sigma-Aldrich), the COS-7 cell line (ATCC), anti-Tmod2 (1:200 for immunocytochemistry and 1:3,000 for western blot, Abcam, Cat # ab67407), anti-complexin-1 and -2 antibody (1:500 for immunocytochemistry and 1:3,000 for western blot, Synaptic Systems, Cat # 122002), anti-HA antibody (1:1,000, Covance, Cat # MMS-101P), anti-Myc antibody (1:1,000, CalBiochem, Cat # OP10), anti-digoxigenin-POD antibody (1:100, Roche, Cat # 11207733910) and anti-actin antibody (1:5,000, Sigma-Aldrich, Cat # A4700). Construction of miRNA sequencing libraries and deep sequencing CA1 regions of mouse hippocampi were removed and homogenized with a Polytron homogenizer (Kinematica) in the lysis buffer provided by the mirVana miRNA Isolation Kit (Ambion). The lysate was extracted with acid-phenol:chloroform, ethanol was added to bring up the sample to 25% and fractionated to isolate the large and small RNAs by using the glass–fiber filter of mirVana miRNA Isolation Kit. RNA integrity number of the extracted RNA samples was measured to assess RNA quality by using the Agilent 2100 Bioanalyzer. miRNAs were purified from the small RNA fraction by using denaturing polyacrylamide gel electrophoresis (15%) followed by recovering the 17–27-nt-long RNA fragments that were enriched for miRNAs. Deep-sequencing libraries were constructed by using the Small RNA Sample Prep kit (Illumina). Briefly, 3′ adaptors and 5′ adaptors were ligated to purified miRNAs sequentially. Adaptor tagged miRNAs were reverse-transcribed and amplified by low-cycle PCR. The PCR products were purified by polyacrylamide gel electrophoresis (8%) and sequenced using an Illumina Genome Analyzer II. Deep-sequencing data analysis Sequence data analysis was performed as previously described [27] . Briefly, raw sequence reads were first consolidated by clustering identical sequence reads. Only reads containing complete 3′ and 5′ adaptor sequences were subjected to downstream analysis. After trimming of 3′ and 5′ adaptor sequences, the remaining sequences were aligned to miRNA hairpin sequences downloaded from the miRBase database ( http://www.mirbase.org/ ) by using Bowtie v0.2.1 (ref. 66 ). Mappable reads were further filtered to remove those that do not map to mature miRNAs. The expression count of each miRNA (≥5 read counts in at least 50% samples) was normalized to the total number of mapped reads of the corresponding sample [67] . The read count was log2-transformed and quantile-normalized across all samples. A modified t -test [68] and FDR analysis [28] were applied to identify differentially expressed miRNAs ( P <0.05). miR-gene-GO enrichment analysis miR-gene-GO enrichment analysis contains three steps (target prediction, target enrichment and GO term enrichment) as described previously [27] . In the first step, the target genes of differentially expressed miRNAs were predicted by using the target prediction tools TargetScan ( http://www.targetscan.org/ ) and miRanda ( http://www.microrna.org/microrna/home.do ). Only target genes predicted by both TargetScan and miRanda were used in the next step of analysis. In the second step, the statistical significance of enrichment for each target gene identified in the first step was determined by using the hypergeometric test, and genes with a P -value <10 −5 were considered significantly enriched. In the last step, GO terms annotating enriched genes identified in the second step were obtained from the Gene Ontology database ( http://www.geneontology.org/ ). As this database is constructed in the directed acyclic graph in which a parent GO term has multiple children terms, GO terms with redundant information are given to genes mapped to both parent and children terms. We therefore used the conditional hypergeometric test, which removes the redundancy for the enrichment analysis. GO terms with a P -value <0.05 were considered significantly enriched. Equation 1 was used for the hypergeometric statistical test in the gene enrichment analysis for each test group. n 11 =the number of miRNAs in the test group that target to the gene being tested; n 12 =the number of other detected miRNAs that had the same change direction as those in the test group, and target to the gene being tested, but were not included in the test group because their FDR-controlled P -values were >0.05; n 21 =the number of miRNAs in the group that do not target to the gene being tested; n 22 =the number of other miRNAs that had the same change direction as those in the test group, but do not target to the gene being tested, and were not included in the test group because their FDR-controlled P -values were >0.05. The enriched GO terms that annotate the over-represented genes were identified by using the conditional hypergeometric test (R package GOStats). GO terms whose statistical significance was contributed by their significant children terms were removed in the conditional hypergeometric test. GO terms that had P -values <0.05 and were targeted by at least 50% of the total selected miRNAs in the test group were considered statistically enriched. Equation 2 was used for the test. There were three sets of GO terms: biological process (BP), molecular function (MF) and cellular component (CC). m 11 =the number of over-represented genes in the test group that were mapped to the GO term being tested; m 12 =the number of other genes in the GO database that were mapped to the GO term being tested; m 21 =the number of over-represented genes in the test group were not mapped to the GO term being tested; m 22 =the number of other genes in the GO database that were not mapped to the GO term being tested. Quantitative reverse transcription PCR miRNAs were purified by using the mirVana miRNA Isolation Kit (Ambion). miRNAs were transcribed into cDNAs and amplified by PCR with the Taqman primers (miR-106b, ID: 442; miR-135a, ID: 460; miR-135b, ID: 2261; miR-136-3p, ID: 2100; miR-19a, ID: 395; miR-19b, ID: 396; miR-191, ID: 2299; miR-466b, ID: 2066; miR-218, ID: 521; miR-29a, ID: 2112; miR-32, ID: 2109) specific for miRNAs of interest. Pri-miRNAs were purified using Trizol (Life technologies), transcribed into cDNAs and amplified by PCR with the primers as follows: miR-191, 5′-AGCTGCACTTGGATTTCGTT-3′ and 5′-TGGCCCAGTAGTGTTTCTGA-3′; miR-135b, 5′-TTCCTGCTCTTTGAGATTCCT-3′ and 5′-GCTGGTCCTTAGGGAAGTGTA-3′; U6, 5′-GCTTCG GCAGCACATATACTAA-3′ and 5′-AAAATATGGAACGCTTCACGA-3′. Applied Biosystems 7900 Fast Real-Time PCR System was used for quantitative reverse transcription PCR. U6 (Taqman probe ID: 1973) was used as the endogenous control gene to normalize input amounts. Neuronal culture and transfection Hippocampal and cortical neuron cultures were prepared from embryonic day (E) 18–19 rat embryos. The hippocampus was removed from the embryo brains, dissociated with trypsin and seeded on coverslips or plates coated with poly- D -lysine (30 μg per ml) and laminin (2 μg per ml) to a density of 750 cells per mm 2 (for spine morphology analysis) or 450 cells per mm 2 (for immunocytochemistry). Cultures were grown in Neurobasal medium supplemented with 2% B27, 2 mM glutamax. Hippocampal neurons were transfected with Lipofectamine 2000. All reagents for neuronal cultures were purchased from Invitrogen. Time-lapse imaging and FRAP Cultured hippocampal neurons were placed in an imaging chamber and perfused with ACSF (composed of (in mM) 124 NaCl, 3 KCl, 26 NaHCO 3 , 1.25 NaH 2 PO 4 , 2.5 CaCl 2 , 1.3 MgSO 4 and 10 D-glucose; bubbled with 95% O 2 /5% CO 2 ; 30 °C) at 2 ml min −1 . Images were acquired by using an Olympus BX61WI confocal microscope with a × 60 objective (NA 1.35). Z-stack images were collapsed to make two-dimensional (2D) projections for image analysis. Spine area and density were analysed by using MetaMorph software (Molecular Devices). Briefly, images were thresholded to remove background. Spines in secondary dendrites were then manually selected and analysed for area and number by using the ‘Integrated Morphometry Analysis’ function of MetaMorph. The length of dendrites was measured by using the ‘Region measurement’ function of MetaMorph. Spine density was calculated by dividing the total number of spines on a given dendrite by the length of the dendrite. Photobleaching of dendrites was performed using the photobleach function of the Olympus Fluoview software. The region of interest was scanned with 100% laser intensity for 30 s followed by normal imaging mode. The integrated SEP intensity of photobleached dendrites at each time point was measured using MetaMorph software, and normalized to that of unbleached dendrites to correct for possible fluorescence decay due to repetitive image acquisition. The proportion of recovered SEP at each time point after bleaching (corrected fluorescence intensity/pre-bleaching fluorescence intensity) was fitted to an exponential curve using the equation F ( t )= F − Ae − t / τ , where F ( t ) is fluorescence at time t , F is the steady state fluorescence after recovery, A is the residual fluorescence after photobleaching and τ is time constant. The image data were analysed with the Kolmogorov–Smirnov and χ 2 test for distribution. As the image data are not normally distributed, two-tailed Mann–Whitney U -test was used to calculate P -values. Immunocytochemistry Hippocampal neurons were fixed in PBS containing 4% formaldehyde and 4% sucrose. After rinse, neurons were incubated with primary antibodies overnight at 4 °C, followed by incubation with fluorophore-conjugated secondary antibodies. Z-stack Images were acquired by using a Zeiss LSM510 confocal microscope with a × 63 (NA 1.4) or × 40 (NA 1.2) objective, and collapsed to make 2D projections. MetaMorph software (Molecular Devices) was used to measure integrated fluorescence intensity of Phalloidin, Tmod2 and complexin-1/2 on the dendrite. All image acquisition and image analysis were done blindly to treatment. The image data were analysed with the Kolmogorov–Smirnov and χ 2 test for distribution. As the image data are not normally distributed, two-tailed Mann–Whitney U -test was used to calculate P -values. Hippocampal slice culture Hippocampal slices were cultured from 6–8-day-old Sprague-Dawley rats. After decapitation, the brain was placed immediately in the cold-cutting solution (238 mM sucrose, 2.5 mM KCl, 26 mM NaHCO 3 , 1 mM NaH 2 PO 4 , 5 mM MgCl 2 , 11 mM D-glucose and 1 mM CaCl 2 ). Hippocampal slices (400 μm) were cut with a vibratome (Leica) and placed on top of semipermeable membrane inserts (Millipore Corporation) in a six-well plate containing culture medium (78.8% minimum essential medium, 20% heat-inactivated horse serum, 25 mM HEPES, 10 mM D-glucose, 26 mM NaHCO 3 , 2 mM CaCl 2 , 2 mM MgSO 4 , 0.0012% ascorbic acid, 1 μg ml −1 insulin; pH 7.3; 320–330 mOsm). Medium was changed every 2 days. No antibiotics were used. Slices were transduced with lentivirus at DIV12 and used for electrophysiology at DIV17. Electrophysiology Hippocampal slices were perfused with artificial cerebrospinal fluid (ACSF, pH 7.4, gassed with 95% O2/5% CO2, composed of in mM: 124 NaCl, 3 KCl, 26 NaHCO3, 1.25 NaH2PO4, 2.5 CaCl2, 1.3 MgSO4 and 10 D -glucose bubbled with 95% O2/5% CO2; 30 °C) at the rate of 2 ml min −1 . The stimulating electrode was placed on the stratum radiatum in the CA2 area. Stimuli were delivered to the electrode at 20 s intervals. Recording pipettes (1–2 MΩ) were filled with the bath solution and placed in the CA1 region. The stimulating electrode was placed at the stratum radiatum in the CA2 area. A 30-min baseline recording was conducted prior to LTD induction. LTD was induced by delivering low-frequency stimulations (900 pulses at 1 Hz). The electrophysiology data were analysed with the Kolmogorov–Smirnov and χ 2 for distribution. As the electrophysiology data are not normally distributed, two-tailed Mann–Whitney U -test was used to calculate P -values. In situ hybridization In situ hybridization of microRNA was performed as described [69] . Briefly, hippocampal neurons were fixed in PBS containing 4% formaldehyde and 4% sucrose. After permeabilization with PBS/0.5% Triton X-100, neurons were hybridized with 5′ and 3′ digoxigenin-labelled, locked nucleic acid-modified oligonucleotide probes (Exiqon) for detection of miRNAs or in vitro -transcribed, digoxigenin-labelled RNAs for detection of mRNAs. Hybridized probes were detected by incubation with horseradish peroxidase-conjugated anti-digoxigenin antibody (Roche) followed by amplification with Cy5-conjugated tyramide (Perkin Elmer). Crosslinking and immunoprecipitation assay Cultured cortical neurons grown on 10 cm dishes were transduced with lentivirus-expressing Flag-tagged Ago2 at DIV 7, and treated with NMDA at DIV 17. Crosslinking and immunoprecipitation of Ago2-associated RNA was performed as described with modifications [70] . At 90 min after NMDA treatment, neurons were crosslinked with UV irradiation (480,000 μJ c −1 m −2 ), and then lysed in 1 × RIPA buffer containing 0.1 U μl −1 RNase inhibitor followed by sonication. After centrifugation at 13,000 r.p.m. for 30 min at 4 °C, supernatant was incubated with anti-Flag antibody-conjugated beads (Sigma-aldrich) overnight with rotation at 4 °C. The beads were washed five times with immunoprecipitation buffer (25 mM HEPES (PH7.5), 150 mM NaCl, 0.5 mM EDTA, 1 mM EGTA, 10% glycerol, 0.1% NP40, 1 mM NaF, 1 mM 2-glycerophosphate, 1 mM Na3VO4). Bound RNAs were extracted with phenol/chloroform, precipitated with ethanol and analysed by qRT–PCR. Accession Codes: The miRNA sequencing data were deposited in the NIH Sequence Read Archive (SRA) database under accession code SRP034860 . How to cite this article: Hu, Z. et al. miR-191 and miR-135 are required for long-lasting spine remodelling associated with synaptic long-term depression. Nat. Commun. 5:3263 doi: 10.1038/ncomms4263 (2014).